miR-1269 promotes metastasis and forms a positive feedback loop with TGF-β As patient survival drops precipitously from early-stage cancers to late-stage and metastatic cancers, microRNAs that promote relapse and metastasis can serve as prognostic and predictive markers as well as therapeutic targets for chemoprevention. Here we show that miR-1269a promotes colorectal cancer (CRC) metastasis and forms a positive feedback loop with TGF-β signalling. miR-1269a is upregulated in late-stage CRCs, and long-term monitoring of 100 stage II CRC patients revealed that miR-1269a expression in their surgically removed primary tumours is strongly associated with risk of CRC relapse and metastasis. Consistent with clinical observations, miR-1269a significantly increases the ability of CRC cells to invade and metastasize in vivo . TGF-β activates miR-1269 via Sox4, while miR-1269a enhances TGF-β signalling by targeting Smad7 and HOXD10, hence forming a positive feedback loop. Our findings suggest that miR-1269a is a potential marker to inform adjuvant chemotherapy decisions for CRC patients and a potential therapeutic target to deter metastasis. Many solid tumours progress through stages while accumulating genetic alterations and reprogramming microenvironments [1] , [2] . Ranked among the most common cancers and a leading cause of cancer-related deaths [3] , [4] , colorectal cancer (CRC) progresses through an adenomas to carcinoma sequence that eventually leads to metastasis [5] , [6] . The stage of CRC is specified by the American Joint Committee on Cancer (AJCC) tumour-node-metastasis staging system, which provides the guideline for treatment. Stages I and II are usually considered non-invasive, stage III has spread to lymph nodes and stage IV involves metastasis. However, although there is consensus to treat stage I CRC with only surgery and stages III/IV CRC with chemotherapy in addition to surgery, the overall benefit of adjuvant chemotherapy after resection of stage II CRC remains unclear [7] . Still, chemotherapy likely improves survival for certain subsets of stage II patients. As patient survival drops from 80 to 90% for early-stage CRCs to below 10% for late-stage and metastatic CRCs, it is important to identify prognostic markers and therapeutic targets for chemoprevention [8] . microRNAs are small noncoding RNA molecules that suppress gene expression via the 3′ untranslated regions (UTRs) of target mRNAs. Individual microRNA can control many target genes and microRNA expression is often altered in cancer cells [9] . Among them, microRNAs that promote relapse and metastasis are of particular interest as potential prognostic biomarkers and therapeutic targets [10] , [11] . In this study, we show that miR-1269a expression is upregulated in late-stage CRC and is associated with recurrence and metastasis of disease-free stage II CRC patients. miR-1269a promotes CRC cells to undergo epithelial–mesenchymal transition (EMT) and to metastasize in vivo . Mechanistically, miR-1269 targets Smad7 and HOXD10 to enhance transforming growth factor (TGF)-β signalling, which in turn upregulates miR-1269 via Sox4. miR-1269 is upregulated in late-stage CRC tumours To investigate the roles of microRNAs in CRC progression, we systematically compared microRNA expression levels in early- versus late-stage CRC tumours using the latest COlon ADenocarcinoma (COAD) miRNASeq data set in The Cancer Genome Atlas (TCGA) [12] (see Methods). Differential expression analysis based on read counts identified miR-1269 as a top microRNA candidate that is upregulated in stage IV CRCs versus stage I and II CRCs, with a P -value of 0.01 ( Fig. 1a–c and Supplementary Fig. 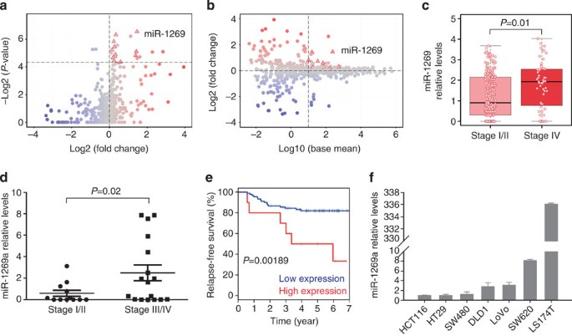Figure 1: miR-1269 level is associated with CRC progression, relapse and metastasis. (a) Volcano plot comparing miRNASeq data between Stage I/II CRCs and Stage IV CRCs from the TCGA COAD data set. Each dot represents a microRNA. Dots in the upper right quadrant represent microRNAs that are upregulated in Stage IV CRCs with enough statistical significance (P-value<0.05 based on DESeq). (b) MA plot comparing miRNASeq data between Stage I/II CRCs and Stage IV CRCs. Dots in the upper right quadrant represent microRNAs that are abundant and upregulated in Stage IV CRCs. (c) miR-1269 expression in early- (Stage I/II,n=230) and late-stage (Stage IV,n=59) CRCs. Each dot represents a CRC sample from COAD. (d) RT–qPCR measurements of miR-1269a expression in early- (Stage I/II,n=12) and late-stage (Stage III/IV,n=17) CRC samples from WCMC Colon Cancer Biobank.P-value was calculated based on Student’st-test. (e) Kaplan–Meier analysis of relapses of Stage II CRC patients with high (red,n=10) and low (blue,n=90) miR-1269a levels in their surgically removed primary tumours. (f) RT–qPCR measurements of miR-1269a expression in various CRC lines. Error bars denote s.d. of triplicates. 1 , Supplementary Table 1 ). We did not include Stage III CRCs in our TCGA analysis because their metastatic potential was less clear and may vary widely between individuals. Figure 1: miR-1269 level is associated with CRC progression, relapse and metastasis. ( a ) Volcano plot comparing miRNASeq data between Stage I/II CRCs and Stage IV CRCs from the TCGA COAD data set. Each dot represents a microRNA. Dots in the upper right quadrant represent microRNAs that are upregulated in Stage IV CRCs with enough statistical significance ( P -value<0.05 based on DESeq). ( b ) MA plot comparing miRNASeq data between Stage I/II CRCs and Stage IV CRCs. Dots in the upper right quadrant represent microRNAs that are abundant and upregulated in Stage IV CRCs. ( c ) miR-1269 expression in early- (Stage I/II, n =230) and late-stage (Stage IV, n =59) CRCs. Each dot represents a CRC sample from COAD. ( d ) RT–qPCR measurements of miR-1269a expression in early- (Stage I/II, n =12) and late-stage (Stage III/IV, n =17) CRC samples from WCMC Colon Cancer Biobank. P -value was calculated based on Student’s t -test. ( e ) Kaplan–Meier analysis of relapses of Stage II CRC patients with high (red, n =10) and low (blue, n =90) miR-1269a levels in their surgically removed primary tumours. ( f ) RT–qPCR measurements of miR-1269a expression in various CRC lines. Error bars denote s.d. of triplicates. Full size image The miR-1269 family has two isoforms, miR-1269a and miR-1269b. 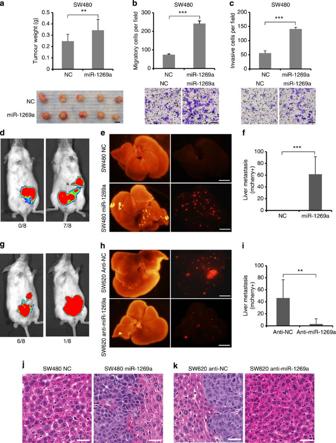Figure 2: miR-1269a promotes CRC metastasis. (a) Growth of subcutanous xenograft CRC tumour, as shown by tumour weight (upper panel) and representative tumour images (lower panel), with a control vector (NC) or with ectopic miR-1269a expression (miR-1269a). Error bars denote s.d. of five mice in each group. Scale bar, 5 mm. (b,c) Transwell assay measuring CRC cell migration (b) and invasion (c) with a control vector (NC) or with ectopic miR-1269a expression (miR-1269a). Error bars denote s.d. of triplicates. Scale bar, 50 μm. (d–f) Analysis of CRC liver metastasis in mice with orthotopic (cecal) injection of SW480-NC and SW480-miR-1269a cells carrying luciferase and mCherry reporter constructs. Representative IVIS luciferasein vivoimages (d), bright field and fluorescent (mCherry) images of livers isolated from mice (e) and number of liver metastatic nodules (f) show ectopic miR-1269a expression-promoted liver metastasis of SW480 cells. Scale bar, 8mm. (g–i) Analysis of CRC liver metastasis in mice with orthotopic (cecal) injection of SW620-Anti-NC and SW620-Anti-miR-1269a cells carrying luciferase and mCherry reporter constructs. Representative IVIS luciferasein vivoimages (g), bright field and fluorescent (mCherry) images of livers (h) and number of liver metastatic nodules (i) show knockdown of endogenous miR-1269a by antisense RNA suppressed liver metastasis of SW620 cells. Error bars denote s.d. of eight mice in each group. Scale bar, 8 mm. (j,k) H&E staining of liver sections isolated from mice orthotopically injected with SW480-NC or SW480-miR-1269a cells (j) or SW6200-Anti-NC or SW620-Anti-miR-1269a cells (k). Error bars denote s.d. of eight mice in each group. Scale bar, 15 μm. **P<0.01; ***P<0.001. Student’st-test. To validate the TCGA analysis, we measured miR-1269a and miR-1269b expression levels in 12 early-stage and 17 late-stage CRC tumours acquired from the Weill Cornell Medical College (WCMC) Colon Cancer Biobank ( Supplementary Table 2 ). Late-stage CRCs have higher miR-1269a expression levels than early-stage CRCs in a statistically significant manner according to reverse transcription–quantitative PCR (RT–qPCR) measurements, consistent with the TCGA finding ( Fig. 1d ). On the other hand, miR-1269b level was not statistically different between early- and late-stage CRC samples. miR-1269 is a marker for CRC relapse and metastasis Generally, it is difficult to predict whether stage II CRC patients will relapse or develop metastasis after surgical removal of their primary tumours, although 10–20% of stage II patients will eventually relapse. To explore whether miR-1269a is a prognostic marker for relapse and metastasis, we performed a clinical study on 100 stage II CRC patients at the Catalan Institute of Oncology ( Tables 1 and 2 ) [13] . These disease-free patients were considered ‘low-risk’ for relapse and did not undergo chemotherapy after the surgery. The patients were divided into two cohorts, ‘miR-1269a low ’ and ‘miR-1269a high ’, based on the miR-1269a expression levels measured in their surgically removed primary tumours. Based on risk of relapse for stage II CRC, we allocated the top 10% (10 patients) into the miR-1269a high cohort and the rest (90 patients) into the miR-1269a low cohort to see whether miR-1269a expression could distinguish the small subset of patients who actually had high risk of relapse. Table 1 Relationship between miR-1269a and clinicopathological features of 100 stage II CRC patients. Full size table Table 2 Multivariate analysis of miR-1269a prognosis. Full size table Follow-up revealed that high miR-1269a expression was associated with relapse and metastasis of these disease-free patients (logrank P =0.002). The miR-1269a high cohort had a significantly higher recurrence rate than the miR-1269a low cohort, based on disease-free survival curves from Kaplan–Meier analysis ( Fig. 1e ). Distant metastasis developed in only 18% of the patients in the miR-1269a low cohort, but in 60% of the patients in the miR-1269a high cohort ( Table 1 ). The prognostic value of miR-1269a for disease-free survival was significant ( P =0.015) in a multivariable Cox’ proportional hazards model adjusted for age, sex, subsite (left/right) and sub-stage (IIa/IIb; Table 2 ). These results indicate that miR-1269a could be a potential marker associated with a small subset of high-risk CRC Stage II patients who were previously deemed low-risk and may benefit from chemotherapy after surgery. We also explored cut points of miR-1269a expression that stratified patients at 15 and 20 upper percentiles, and the miR-1269a high cohort still had higher recurrence rate than the miR-1269a low cohort in a statistically significant way ( P =0.009 and 0.022). Similar analysis on miR-1269b showed that miR-1269b was not associated with risk of relapse ( Supplementary Fig. 2a ). miR-1269a expression in CRC cell lines We measured miR-1269a expression in six commonly used CRC cell lines ( Fig. 1f ). In general, miR-1269a levels are low in cells with relatively low metastatic potential (HT29 and SW480), and are high in cells with relatively high metastatic potential (DLD1, LoVo, LS174T and SW620). One ambivalent case is the low miR-1269a expression in HCT116 cells, which were derived from primary adenocarcinoma but seem to possess metastatic potential. It is likely that HCT116 cells have accumulated other metastasis-promoting mutations. Notably, the miR-1269a level is sixfold higher in SW620 cells than in SW480 cells. Originally from the same CRC patient, SW480 was derived from a primary colon adenocarcinoma before relapse, whereas SW620 was derived from mesenteric lymph nodes metastases post-relapse [14] . Hence, this controlled comparison between the two patient-matched cell lines supported that miR-1269a levels are associated with metastatic potential. Unlike miR-1269a, miR-1269b exhibited similar expression levels in SW480 and SW620 cells ( Supplementary Fig. 2b ). Therefore, we decided to focus on miR-1269a for the rest of the study. miR-1269a promotes CRC metastasis To evaluate the effect of miR-1269a on SW480 cells, which have low endogenous miR-1269a expression, we ectopically expressed miR-1269a in SW480 cells. Ectopic miR-1269a only slightly increased cell growth in vitro ( Supplementary Fig. 3 ) and subcutaneous xenograft tumour growth in vivo ( Fig. 2a ). However, Transwell migration assay ( Fig. 2b ) and Matrigel invasion assay ( Fig. 2c ) showed that ectopic expression of miR-1269a increased migration and invasion of SW480 cells significantly. Figure 2: miR-1269a promotes CRC metastasis. ( a ) Growth of subcutanous xenograft CRC tumour, as shown by tumour weight (upper panel) and representative tumour images (lower panel), with a control vector (NC) or with ectopic miR-1269a expression (miR-1269a). Error bars denote s.d. of five mice in each group. Scale bar, 5 mm. ( b , c ) Transwell assay measuring CRC cell migration ( b ) and invasion ( c ) with a control vector (NC) or with ectopic miR-1269a expression (miR-1269a). Error bars denote s.d. of triplicates. Scale bar, 50 μm. ( d – f ) Analysis of CRC liver metastasis in mice with orthotopic (cecal) injection of SW480-NC and SW480-miR-1269a cells carrying luciferase and mCherry reporter constructs. Representative IVIS luciferase in vivo images ( d ), bright field and fluorescent (mCherry) images of livers isolated from mice ( e ) and number of liver metastatic nodules ( f ) show ectopic miR-1269a expression-promoted liver metastasis of SW480 cells. Scale bar, 8mm. ( g–i ) Analysis of CRC liver metastasis in mice with orthotopic (cecal) injection of SW620-Anti-NC and SW620-Anti-miR-1269a cells carrying luciferase and mCherry reporter constructs. Representative IVIS luciferase in vivo images ( g ), bright field and fluorescent (mCherry) images of livers ( h ) and number of liver metastatic nodules ( i ) show knockdown of endogenous miR-1269a by antisense RNA suppressed liver metastasis of SW620 cells. Error bars denote s.d. of eight mice in each group. Scale bar, 8 mm. ( j , k ) H&E staining of liver sections isolated from mice orthotopically injected with SW480-NC or SW480-miR-1269a cells ( j ) or SW6200-Anti-NC or SW620-Anti-miR-1269a cells ( k ). Error bars denote s.d. of eight mice in each group. Scale bar, 15 μm. ** P <0.01; *** P <0.001. Student’s t -test. Full size image To investigate whether miR-1269a promotes metastasis in vivo , we used an established CRC orthotopic model by implanting human CRC cells into cecum terminus of NOD/SCID mice [15] , [16] . SW480 cells were infected with lentiviral vectors to establish two stable lines that either expressed miR-1269a (SW480-miR-1269a) or contained a control vector (SW480-NC). These cells also carry constitutive luciferase and mCherry reporter constructs. After cecal implantation of equal numbers of cells from both lines, metastasis was tracked using the whole-body IVIS bioluminescence imaging system. Once a mouse became moribund, all mice were killed simultaneously and hepatic metastases expressing mCherry were analysed by imaging the entire liver with a fluorescent microscope. SW480-NC cells failed to metastasize to liver in all 8 mice (0/8). In contrast, 7 out 8 (7/8) mice injected with SW480-miR-1269a cells developed hepatic metastases ( Fig. 2d,e,f,j and Supplementary Fig. 4a,b ). Hence, ectopic miR-1269a expression promotes metastasis of SW480 cells in vivo . To investigate whether silencing of miR-1269a expression in metastatic cells impedes their ability to metastasize, we knocked down endogenous miR-1269a levels in SW620 cells, the metastatic counterpart of SW480 from the same patient. SW620 cells were infected with lentiviral vectors to establish two stable lines that either expressed antisense RNA against miR-1269a (SW620-Anti-miR-1269a) or contained a control vector (SW620-Anti-NC). The mir-1269a knockdown efficiency in SW620-Anti-miR-1269a cells was evaluated by a luciferase reporter ( Supplementary Fig. 5 ). Equal numbers of SW620-Anti-NC and SW620-Anti-miR-1269a cells were implanted into the ceca of NOD/SCID mice. All mice were simultaneously killed for metastasis examination when one became moribund. Six out of eight (6/8) mice injected with SW620-Anti-NC cells developed hepatic metastases, whereas only 1 out of 8 (1/8) mice injected with SW620-Anti-miR-1269a cells developed hepatic metastasis ( Fig. 2g,h,i,k and Supplementary Fig. 4c,d ). Thus, miR-1269a knockdown suppressed metastasis of SW620 cells in vivo . In addition to the cecum-injection model, we performed intravenous injection through tail vein with the same cells. In the group injected with SW480-miR-1269 cells, all 10 mice developed lung metastasis, with a large number of metastatic nodules covering the entire lung. In contrast, only 4 out of 10 mice injected with SW480-NC cells developed lung metastasis, with a small number of metastatic nodules ( Supplementary Fig. 6a–c ). miR-1269a also promoted CRC colonization of the liver. Only 1 out of the 10 mice injected with SW480-NC cells developed liver metastasis, whereas 5 out of the 10 mice injected SW480-miR-1269a cells developed liver metastasis ( Supplementary Fig. 6d-f ). Consistent with SW480 cells, ectopic miR-1269a expression in HCT116 also enhanced lung and liver metastasis, compared with the control vector ( Supplementary Fig. 6g,h ). Therefore, miR-1269a expression promoted colonization of circulating SW480 and HCT116 cells in the lung and the liver. Similarly, equal numbers of SW620-Anti-NC and SW620-Anti-miR-1269a were intravenously injected through tail vein. In the control group (SW620-Anti-NC), all 10 mice (10/10) developed lung metastasis and 4 out of 10 (4/10) developed liver metastasis, which is consistent with the high metastatic potential of SW620. miR-1269a knockdown significantly reduced lung and liver metastasis of SW620 cells. In the SW620-Anti-miR-1269a group, only 3 out 10 (3/10) mice developed lung metastasis and 1 out 10 (1/10) developed liver metastasis ( Supplementary Fig. 6a–f ). The SW620 data were further corroborated by knocking down miR-1269a in LS174T cells, which also have high endogenous miR-1269a expression. Injected LS174T control cells formed extensive metastasis in the lung, lymph nodes in the lateral thoracic region and the bone. In contrast, miR-1269a knockdown in LS174T cells significantly reduced metastasis in these regions ( Supplementary Fig. 6i ). Therefore, silencing of endogenous miR-1269a mitigated colonization of circulating SW620 and LS174T cells. Collectively, the in vitro migration and invasion assays and in vivo metastasis assays, with ectopic expression of miR-1269a in SW480 and HCT116 cells and knockdown of endogenous miR-1269a in SW620 and LS174T cells, indicate that miR-1269a promotes CRC metastasis. miR-1269a promotes an EMT-like process As an EMT-like process has been associated with colon cancer metastasis [17] , we examined whether miR-1269a promotes EMT. We measured the levels of the epithelial marker E-cadherin and the mesenchymal markers N-cadherin and Vimentin in SW480-miR-1269a and SW480-NC cells using both western blot analysis and immunofluorescence. Compared with the control SW480-NC cells, which had high E-cadherin expression and low N-cadherin and Vimentin expression, SW480-miR-1269a cells had significantly downregulated E-cadherin expression and upregulated N-cadherin and Vimentin expression ( Fig. 3a,b ). Consistent with the EMT markers, SW480-miR-1269a cells adopted a spindle-shaped, mesenchymal-like morphology in contrast to the epithelial-like morphology of SW480-NC cells ( Fig. 3c ). Hence ectopic miR-1269a expression causes SW480 cells to undergo EMT. 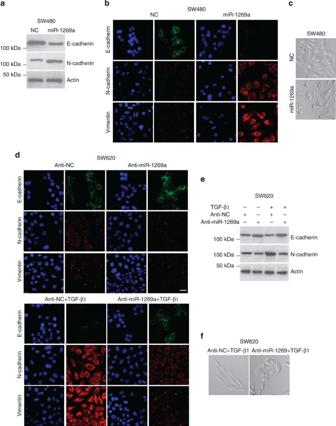Figure 3: miR-1269a regulates EMT. (a–c) Western blot (a), immunofluorescence (b) and phase-contract images (c) of SW480 cells with a control vector (NC) or with ectopic miR-1269a expression (miR-1269a). Ectopic miR-1269a downregulated the epithelial marker E-cadherin, upregulated the mesenchymal markers N-cadherin and Vimentin, and changed cell morphology. (d–f) Immunofluorescence (d), western blot (e) and phase-contract images (f) of SW620 cells with a control vector (Anti-NC) or with antisense RNA against endogenous miR-1269a (Anti-miR-1269a). SW620 cells are either untreated (d, upper panel) or treated with TGF-β1 (d, lower panel). miR-1269a knockdown suppressed TGF-β1 induction of EMT, as indicated by downregulation of N-cadherin and Vimentin, upregulation of E-cadeherin, and reversion from a mesenchymal-like morphology to an epithelial-like morphology. Scale bar, 15 μm. Figure 3: miR-1269a regulates EMT. ( a – c ) Western blot ( a ), immunofluorescence ( b ) and phase-contract images ( c ) of SW480 cells with a control vector (NC) or with ectopic miR-1269a expression (miR-1269a). Ectopic miR-1269a downregulated the epithelial marker E-cadherin, upregulated the mesenchymal markers N-cadherin and Vimentin, and changed cell morphology. ( d–f ) Immunofluorescence ( d ), western blot ( e ) and phase-contract images ( f ) of SW620 cells with a control vector (Anti-NC) or with antisense RNA against endogenous miR-1269a (Anti-miR-1269a). SW620 cells are either untreated ( d , upper panel) or treated with TGF-β1 ( d , lower panel). miR-1269a knockdown suppressed TGF-β1 induction of EMT, as indicated by downregulation of N-cadherin and Vimentin, upregulation of E-cadeherin, and reversion from a mesenchymal-like morphology to an epithelial-like morphology. Scale bar, 15 μm. Full size image We then examined whether silencing of miR-1269a could impede the ability of cells to undergo EMT. As the metastatic counterpart of SW480, SW620 cells have higher endogenous miR-1269a expression levels than SW480 cells. miR-1269a knockdown reduced N-cadherin and Vimentin levels in SW620 cells, as shown by immunofluorescence and western blot ( Fig. 3d,e ). TGF-β1 treatment turned on N-cadherin and Vimentin expression and turned down E-cadherin expression in the control (SW620-Anti-NC) cells, which started to display a mesenchymal-like morphology ( Fig. 3f ). In contrast, the effect of TGF-β1 induction was much attenuated by miR-1269a knockdown, as SW620-Anti-miR-1269a cells largely maintained E-cadherin expression and the epithelial-like morphology in the presence of TGF-β1 ( Fig. 3d–f ). Therefore, miR-1269a knockdown impedes the ability of SW620 cells to undergo an EMT-like process upon TGF-β induction. Together, the data indicate that miR-1269a not only promotes an EMT-like process, but is also involved with TGF-β-induced transformation of CRC cells. TGF-β activates miR-1269a via Sox4 To explore the crosstalk between miR-1269a and TGF-β, we treated SW480 cells with TGF-β1 and measured the response of miR-1269a by RT–qPCR. TGF-β1 treatment upregulated miR-1269a expression, suggesting that TGF-β is an upstream regulator of miR-1269a ( Fig. 4a ). Genomic analysis identified two Sox4-binding motifs at −173 to −166 (site 1) and −947 to −940 (site 2) inside the putative miR-169 promoter region ( Fig. 4b ). Notably, Sox4 is a downstream target gene of TGF-β [18] and has been reported to be a master regulator of EMT and cancer metastasis [19] . Therefore, Sox4 is a potential intermediate between TGF-β and miR-1269a. Notably, Sox4 expression level was higher in SW620 cells than in SW480 cells, similar to miR-1269 ( Supplementary Fig. 7 ). 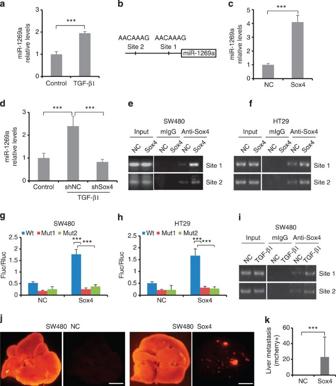Figure 4: Sox4 activates miR-1269a expression directly. (a) RT–qPCR showing TGF-β1 treatment induces miR-1269a expression in SW480 cells. (b) A schematic diagram illustrating the two putative Sox4 binding sites in the miR-1269a promoter. (c) RT–qPCR showing ectopic Sox4 expression upregulates miR-1269a expression in SW480 cells. (d) RT–qPCR showing Sox4 knockdown by an short hairpin RNA (shRNA) abolishes TGF-β1 induction of miR-1269a. (e,f) ChIP assay of SW480 (e) and HT29 (f) cells infected with a control (NC) or a Sox expression (Sox4) vector. Binding of Sox4 to the two sites was confirmed by PCR with primers specific for the two sites. (g,h) Luciferase reporter assays confirming Sox4 activation of the miR-1269a promoter through the two Sox4-binding sites in SW480 (g) and HT29 (h) cells. Expression of firefly luciferase (Fluc) was driven by miR-1269a promoter sequences containing either wild-type (Wt) or mutated (Mut1, Mut2) Sox4-binding sites. Ectopic expression of Sox4 upregulates luciferase in Wt cells, but not in Mut1 and Mut2 cells. Fluc signals were normalized by a simultaneously delivered Renillar luciferase (Rluc) expression plasmid. (i) ChIP assay of SW480 cells treated with TGF-β1. Sox4 binding to the two sites was confirmed by PCR with primers specific for the two sites. (j,k) Bright field and fluorescent (mCherry) images of livers isolated from mice orthotopically injected with SW480-NC and SW480-Sox4 cells (j), and number of liver metastatic nodules. Ectopic Sox4 expression promoted liver metastasis of SW480 cells. Error bars inkdenote s.d. of each group (8 mice). Scale bar, 8 mm. In remaining cases, error bars denote s.d. of triplicates. ***P<0.001, Student’st-test. Figure 4: Sox4 activates miR-1269a expression directly. (a ) RT–qPCR showing TGF-β1 treatment induces miR-1269a expression in SW480 cells. ( b ) A schematic diagram illustrating the two putative Sox4 binding sites in the miR-1269a promoter. ( c ) RT–qPCR showing ectopic Sox4 expression upregulates miR-1269a expression in SW480 cells. ( d ) RT–qPCR showing Sox4 knockdown by an short hairpin RNA (shRNA) abolishes TGF-β1 induction of miR-1269a. ( e , f ) ChIP assay of SW480 ( e ) and HT29 ( f ) cells infected with a control (NC) or a Sox expression (Sox4) vector. Binding of Sox4 to the two sites was confirmed by PCR with primers specific for the two sites. ( g,h ) Luciferase reporter assays confirming Sox4 activation of the miR-1269a promoter through the two Sox4-binding sites in SW480 ( g ) and HT29 ( h ) cells. Expression of firefly luciferase (Fluc) was driven by miR-1269a promoter sequences containing either wild-type (Wt) or mutated (Mut1, Mut2) Sox4-binding sites. Ectopic expression of Sox4 upregulates luciferase in Wt cells, but not in Mut1 and Mut2 cells. Fluc signals were normalized by a simultaneously delivered Renillar luciferase (Rluc) expression plasmid. ( i ) ChIP assay of SW480 cells treated with TGF-β1. Sox4 binding to the two sites was confirmed by PCR with primers specific for the two sites. ( j , k ) Bright field and fluorescent (mCherry) images of livers isolated from mice orthotopically injected with SW480-NC and SW480-Sox4 cells (j), and number of liver metastatic nodules. Ectopic Sox4 expression promoted liver metastasis of SW480 cells. Error bars in k denote s.d. of each group (8 mice). Scale bar, 8 mm. In remaining cases, error bars denote s.d. of triplicates. *** P <0.001, Student’s t -test. Full size image We then tested whether Sox4 can activate the miR-1269a promoter as suggested by their binding motifs. In SW480 cells, ectopic expression of Sox4 caused a fourfold increase of miR-1269a expression level, compared with cells transfected with a control vector ( Fig. 4c ). We then tested whether Sox4 is the intermediate regulator that is required for TGF-β-induced miR-1269a upregulation. Compared with the control cells, Sox4 knockdown by short hairpin RNA (shSox4) completely abolished the effect of TGF-β1 on miR-1269a expression, consistent with Sox4 as an intermediate regulator between TGF-β1 and miR-1269a ( Fig. 4d ). To address whether Sox4 directly activates miR-1269a expression, we performed chromatin immunoprecipitation (ChIP) assays in SW480 and HT29 cells. ChIP confirmed that Sox4 proteins were recruited to both binding sites in the putative miR-1269a promoter, with the majority of Sox4 bound to site 1 ( Fig. 4e, f ). To test whether the binding of Sox4 is sufficient to activate miR-1269a expression, we cloned the putative miR-1269a promoter sequence into a pGL4-basic vector, which were subsequently transfected into SW480 and HT29 cells. A dual-luciferase reporter assay revealed that ectopic expression of Sox4 activated the transcription of firefly luciferase that was driven by the wild-type miR-1269a promoter. When the binding sequence of site 1 was mutated, firefly luciferase expression dropped 6.8-fold in SW480 cells and 5.4-fold in HT29. When the binding sequence of site 2 was mutated, firefly luciferase expression dropped 4.6-fold in SW480 and 5.7-fold in HT29 ( Fig. 4g, h ). Therefore, Sox4 directly binds to these two sites to activate miR-1269a expression. We then examined whether endogenous Sox4 binding to the miR-1269 promoter increases upon TGF-β induction. We treated SW480 cells with TGF-β1 and then performed ChIP. As expected, more Sox4 proteins were recruited to both binding sites in the miR-1269 promoter after TGF-β1 treatment ( Fig. 4i ). Next, to investigate whether Sox4 promotes in vivo metastasis as miR-1269 does, we ectopically expressed Sox4 in SW480 cells and implanted them into mouse ceca. Consistent with ectopic miR-1269 expression, ectopic Sox4 expression significantly enhanced SW480 hepatic metastasis ( Fig. 4j,k ). Taken together, our data indicate that TGF-β upregulates miR-1269a through Sox4, which binds to the two Sox4-binding sites in the miR-1269a promoter to activate miR-1269a expression. Thus, TGF-β, Sox4 and miR-1269a act synergistically to promote EMT and metastasis. miR-1269a targets Smad7 and HOXD10 To determine miR-1269a target genes, we searched for computationally predicted candidates using miRecords, which compiles 11 microRNA targets prediction databases such as PicTar, miRanda, TargetScan and RNA hybrid ( Supplementary Table 3 ). We then used RT–qPCR to compare expression levels of the candidate genes between ectopic miR-1269a expression and control in SW480 and HT29 cells. Among the candidates, homeobox D10 (HOXD10) has been reported to suppress tumour invasion and metastasis [20] , whereas Smad7 is a well-known antagonist of TGF-β signalling [21] . Smad7 and HOXD10 were downregulated in both SW480 and HT29 cells by miR-1269a ( Fig. 5a,b ). Western blot confirmed that miR-1269a suppresses Smad 7 and HOXD10 protein levels ( Fig. 5c,d ). 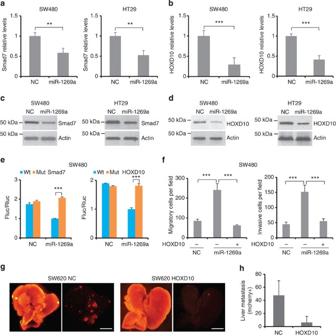Figure 5: HOXD10 and Smad7 are direct targets of miR-1269a. (a,b) RT–qPCR of Smad7 (a) and HOXD10 (b) mRNA levels in SW480 and HT29 cells with a control vector (NC) or with an ectopic miR-1269a expression vector (miR-1269a). (c,d) Western blot of Smad7 (c) and HOXD10 (d) protein levels in SW480 and HT29 cells with a control vector (NC) or with an ectopic miR-1269a expression vector (miR-1269a). (e) Luciferase reporter assays confirming the miR-1269a-binding sites in Smad7 and HOXD10 3′UTRs. 3′UTRs of Smad7 (left) and HOXD10 (right) containing wild-type (Wt) or mutated (Mut) putative miR-1269a-binding sites were cloned into the 3′UTR of firefly luciferase (Fluc). Ectopic miR-1269a expression in SW480 cells downregulated luciferase in Wt cells, but not in Mut cells. Fluc signals were normalized by a simultaneously delivered Renillar luciferase (Rluc) expression plasmid. (f) Transwell migration assay (left) and Matrigel invasion assay (right) of SW480 cells carrying control (NC) or miR-1269a expression (miR-1269a) vectors. Transient expression of HOXD10 abrogated miR-1269a-induced migration and invasion. Error bars denote the s.d. between triplicates. (g,h) Bright field and fluorescent (mCherry) images of livers isolated from mice orthotopically injected with SW620-NC and SW620-HOXD10 cells (j), and number of liver metastatic nodules (h). Ectopic HOXD10 expression reduced liver metastasis of SW620 cells. Error bars inhdenote s.d. of each group (8 mice). Scale bar, 8 mm. In remaining cases, error bars denote s.d. of triplicates. **P<0.01; ***P<0.001, Student’st-test. Figure 5: HOXD10 and Smad7 are direct targets of miR-1269a. ( a , b ) RT–qPCR of Smad7 ( a ) and HOXD10 ( b ) mRNA levels in SW480 and HT29 cells with a control vector (NC) or with an ectopic miR-1269a expression vector (miR-1269a). ( c , d ) Western blot of Smad7 ( c ) and HOXD10 ( d ) protein levels in SW480 and HT29 cells with a control vector (NC) or with an ectopic miR-1269a expression vector (miR-1269a). ( e ) Luciferase reporter assays confirming the miR-1269a-binding sites in Smad7 and HOXD10 3′UTRs. 3′UTRs of Smad7 (left) and HOXD10 (right) containing wild-type (Wt) or mutated (Mut) putative miR-1269a-binding sites were cloned into the 3′UTR of firefly luciferase (Fluc). Ectopic miR-1269a expression in SW480 cells downregulated luciferase in Wt cells, but not in Mut cells. Fluc signals were normalized by a simultaneously delivered Renillar luciferase (Rluc) expression plasmid. ( f ) Transwell migration assay (left) and Matrigel invasion assay (right) of SW480 cells carrying control (NC) or miR-1269a expression (miR-1269a) vectors. Transient expression of HOXD10 abrogated miR-1269a-induced migration and invasion. Error bars denote the s.d. between triplicates. ( g , h ) Bright field and fluorescent (mCherry) images of livers isolated from mice orthotopically injected with SW620-NC and SW620-HOXD10 cells ( j ), and number of liver metastatic nodules ( h ). Ectopic HOXD10 expression reduced liver metastasis of SW620 cells. Error bars in h denote s.d. of each group (8 mice). Scale bar, 8 mm. In remaining cases, error bars denote s.d. of triplicates. ** P <0.01; *** P <0.001, Student’s t -test. Full size image To test whether they are direct targets of miR-1269a, the 3′UTRs of the two genes were cloned downstream of firefly luciferase. The luciferase reporters were then co-transfected with a miR-1269a-expressing construct or an empty control vector into SW480 cells. Cells with ectopic miR-1269a expression had suppressed Smad7 and HOXD10 levels, in contrast to the control cells, whereas mutation in the putative miR-1269a seed regions in the 3′UTRs of either Smad7 or HOXD10 abrogated the suppression of miR-1269a ( Fig. 5e and Supplementary Fig. 8 ). Therefore, miR-1269a directly targets Smad7 and HOXD10 through the identified binding sites in their 3′UTR. HOXD10 has been reported to suppress tumour invasion and metastasis [20] . To test whether miR-1269a suppression of HOXD10 promotes invasion and metastasis, we transfected SW480 cells with vector constructs expressing both miR-1269a and HOXD10 mRNA without its 3′UTR (hence resistant to miR-1269a suppression). Transwell migration and Matrigel invasion assays revealed that ectopic expression of HOXD10 was able to abrogate miR-1269a-induced cell migration and invasion ( Fig. 5f ). We then ectopically expressed HOXD10 in SW620 cells and implanted the cells orthotopically into mouse cecum termini. Consistent with the in vitro migration and invasion assays, ectopic HOXD10 expression dramatically reduced hepatic metastasis in vivo ( Fig. 5g,h ). miR-1269a and TGF-β forms a positive feedback loop Smad7 is a well-known antagonist of TGF-β signalling [21] , although the effect of HOXD10 on TGF-β signalling is unclear. This raised the question as to whether miR-1269a regulates TGF-β signalling in CRC cells through its direct targets. Western blot showed that ectopic expression of miR-1269 in SW480 cells enhanced Smad2 phosphorylation. Consistently, Knockdown of miR-1269 target Smad7 or HOXD10 also promoted Smad2 phosphorylation ( Fig. 6a ). To evaluate the effect of HOXD10 and Smad7 on TGF-β targets gene expression, we established cell lines either expressing Smad7 or HOXD10, or containing a control vector. The cell lines were treated with TGF-β1 for 96 h before RT–qPCR and western blot were performed to measure TGF-β target genes, Slug, Snail and Sox4. As expected, TGF-β1 upregulated Slug, Snail and Sox4 expression in cell lines with the control vector. However, the upregulation was significantly reduced by ectopic expression of Smad7 or HOXD10 ( Fig. 6b–e and Supplementary Fig. 9a–d ), suggesting that HOXD10 is also an antagonist of TGF-β signalling in CRC cells. Ectopic expression of Smad7 or HOXD10 also reduced TGF-β induced miR-1269a upregulation, consistent with the fact that Sox4 levels are down ( Fig. 6f and Supplementary Fig. 9e ). Taken together, these data indicate that Smad7 and HOXD10 are antagonists of TGF-β signalling. 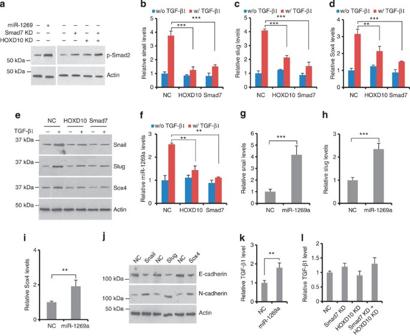Figure 6: miR-1269a upregulates TGF-β signalling by targeting Smad7 and HOXD10. (a) Western blot of phosphorylated Smad2, levels of which were increased by ectopic miR-1269a expression or knockdown of Smad7 or/and HOXD10. (b–e) RT–qPCR and western blot showing ectopic expression of HOXD10 or Smad7 significantly reduced TGF-β1 induction of Snail, Slug and Sox4 expression in SW480. (f) RT–qPCR showing ectopic expression of HOXD10 or Smad7 significantly reduced TGF-β1 induction of miR-1269a in SW480 cells. (g–i) RT–qPCR showing ectopic expression of miR-1269a upregulated Snail, Slug and Sox4 in SW480 cells. (j) Western blot showing ectopic Snail, Slug or Sox4 upregulated E-cadherin and downregulated N-cadherin in SW480 cells. (j) ELISA assay showing that ectoptic miR-1269a expression increased TGF-β1 level in SW480 medium. (k) ELISA assay showing that knockdown of Smad7 and HOXD10 had little effect on TGF-β1 level in SW480 medium. In all case, error bars denote s.d. of triplicates. **P<0.01; ***P<0.001, Student’st-test. w/, with; w/o, without. Figure 6: miR-1269a upregulates TGF-β signalling by targeting Smad7 and HOXD10. ( a ) Western blot of phosphorylated Smad2, levels of which were increased by ectopic miR-1269a expression or knockdown of Smad7 or/and HOXD10. ( b–e ) RT–qPCR and western blot showing ectopic expression of HOXD10 or Smad7 significantly reduced TGF-β1 induction of Snail, Slug and Sox4 expression in SW480. ( f ) RT–qPCR showing ectopic expression of HOXD10 or Smad7 significantly reduced TGF-β1 induction of miR-1269a in SW480 cells. ( g–i ) RT–qPCR showing ectopic expression of miR-1269a upregulated Snail, Slug and Sox4 in SW480 cells. ( j ) Western blot showing ectopic Snail, Slug or Sox4 upregulated E-cadherin and downregulated N-cadherin in SW480 cells. ( j ) ELISA assay showing that ectoptic miR-1269a expression increased TGF-β1 level in SW480 medium. ( k ) ELISA assay showing that knockdown of Smad7 and HOXD10 had little effect on TGF-β1 level in SW480 medium. In all case, error bars denote s.d. of triplicates. ** P <0.01; *** P <0.001, Student’s t -test. w/, with; w/o, without. Full size image As miR-1269a directly targets Smad7 and HOXD10, both of which are antagonists of TGF-β signalling, we examined whether miR-1269a upregulates TGF-β signalling. As showed in Fig. 6g–i and Supplementary Fig. 9f–h , ectopic expression of miR-1269a increased the expression levels of all three target genes of TGF-β signalling, Slug, Snail and Sox4, in SW480 and HT29 cells. Slug, Snail and Sox4 are master regulators of EMT, and their expression in SW480 cells downregulated E-cadherin and upregulated N-cadherin ( Fig. 6j ). These data provide an explanation for the strong induction of EMT by miR-1269a in CRC cells—miR-1269a upregulates TGF-β signalling and its target genes, Slug, Snail and Sox4, via suppression of TGF-β antagonists Smad7 and HOXD10. To examine whether miR-1269a induces TGF-β expression, we performed RT–qPCR in SW480 cells that ectopically express miR-1269a. miR-1269a increased TGF-β1 expression, but had little effect on TGF-β2 and TGF-β3 expression ( Supplementary Fig. 10 ). ELISA confirmed that miR-1269a also increased TGF-β1 protein level in SW480 medium ( Fig. 6k ). miR-1269a seems to upregulate TGF-β1 via a regulatory route independent of Smad7 and HOXD10, as knockdown of Smad7 and HOXD10 did not affect TGF-β1 level ( Fig. 6i ). Our studies suggest that TGF-β and miR-1269a form a positive feedback loop, wherein TGF-β upregulates miR-1269 via Sox4, whereas miR-1269 upregulates TGF-β1 and enhances TGF-β signalling by suppressing its antagonists Smad7 and HOXD10 ( Fig. 7 ). 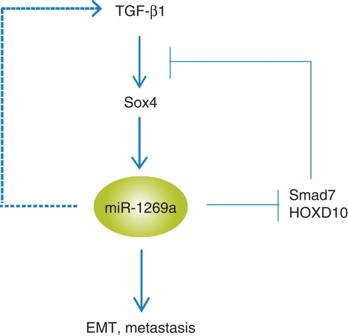Figure 7: A positive feedback loop between TGF-β and miR-1269a. A schematic illustration of the positive feedback loop. miR1269a upregulates TGF-β1 and TGF-β signalling by suppressing its antagonists Smad7 and HOXD10. TGF-β in turn upregulates miR-1269 through Sox4. Figure 7: A positive feedback loop between TGF-β and miR-1269a. A schematic illustration of the positive feedback loop. miR1269a upregulates TGF-β1 and TGF-β signalling by suppressing its antagonists Smad7 and HOXD10. TGF-β in turn upregulates miR-1269 through Sox4. Full size image In this study, we performed differential analysis between early- and late-stage CRCs in TCGA to identify miR-1269 as a top candidate, which was confirmed by additional 29 CRC samples. A study of 100 stage II CRC patients revealed that miR-1269a expression level was associated with risk of relapse and metastasis. Mechanistically, this is because miR-1269a and TGF-β form a positive feedback loop via Sox4, HOXD10 and Smad7 to promote EMT and metastasis. miR-1269a was a somewhat surprising candidate that emerged from our differential analysis because very little was known about this microRNA. A global study of eight paired samples of normal mucosa and CRC tumour reported that miR-1269 was one of the 16 microRNAs that were deregulated in tumour tissues [22] . Nevertheless, a differential expression analysis between normal and tumour tissues in TCGA did not suggest a statistically significant change in miR-1269a expression. Regardless, our analysis suggests that miR-1269a likely plays a more prominent role in CRC relapse and metastasis than in oncogenesis. Hence, the practice of grouping CRC tumours of various stages into a single group may mask the complexity of microRNA regulation during tumour progression. miR-1269a does not promote metastasis alone; instead, it forms a positive feedback loop with TGF-β. This finding is consistent with the increasing appreciation that microRNAs form regulatory motifs with protein regulators to confer robustness to biological processes, and their subversion can expose cells to elevated risk of malfunction [23] . Therefore, the context is important for understanding the role of microRNAs in regulatory networks. For example, positive feedback is known to amplify a response and commits into a self-sustained mode that is autonomous to the original stimuli. It is tempting to speculate that, once induced by TGF-β, the miR-1269a-mediated feedback loop allows CRC cells to become more autonomous. This would enhance the ability of CRC cells to invade and metastasize to new microenvironments, which would explain the strong pro-metastasis phenotype we have observed. Elevated TGF-β production is associated with high risk of CRC relapse and metastasis [24] . Stromal cells in the CRC microenvironment can also produce TGF-β, which increases the efficiency of organ colonization by CRC cells. In a likely scenario, TGF-β released from the microenvironment reaches a certain concentration to activate the positive feedback loop in CRC cells and promote their dissemination. Hence, miR-1269a may play an integrated role in the TGF-β-mediated crosstalk between CRC and stromal cells to confer a survival advantage to metastatic cells. On the other hand, we certainly have to caution against over-simplification of CRC metastasis, which is a complicated process involving many players. In fact, our analysis indicates that, unlike miR-1269a, the association between TGF-β and relapse is not statistically significant among the 100 disease-free stage II CRC patients. This suggests that miR-1269a’s ability to promote recurrence and metastasis does not completely depend on its upregulation of TGF-β in tumour cells. Mutations could interfere with this feedback loop, whereas miR-1269a might also affect metastasis through other targets independent of TGF-β. Neither miR-1269a nor the positive feedback loop is likely to be sufficient or necessary for metastasis. Cell lines Human CRC cell lines SW480, SW620, HCT116, HT29, DLD1, LoVo and LS174T were acquired from American Type Culture Collection and cultured under the conditions recommended by the provider. For TGF-β activation, the cells were treated with 10 ng ml −1 TGF-β1 for 96 h, and TGF-β1 was replaced after 48 h. Kaplan–Meier relapse analysis and clinical specimens The studies followed informed consent and approval of the Ethical Committees at the Catalan Institute of Oncology and Weill Cornell Medical College. Tumour relapse was analysed by tracking 100 stage II CRC patients. The patients were divided into two groups, ‘miR-1269 low ’ and ‘miR-1269 high ’, based on the miR-1269 expression levels measured in their surgically removed primary tumours. microRNA expression was measured using Solid IV small-RNA sequencing and bowtie2 mapped to miRbase 20. Sample counts were normalized according to the library size using the DESeq bioconductor package ( http://genomebiology.com/2010/11/10/r106 ). The cutoff threshold was set to separate the top 10% miR-1269 high patients from the 90% ‘miR-1269 low patients. The disease-free survival curves were estimated using the Kaplan–Meier method and compared with the log-rank test. To evaluate miR-1269a expression in early- and late-stage CRC tumours, frozen CRC specimens were acquired from the WCMC Colon Cancer Biobank. Total RNA was then isolated from the frozen tissues using the Allprep DNA/RNA kit (Qiagen). Quantitative real-time RT–PCR analysis Total RNA was extracted from the cells using the TRIzol Reagent (Invitrogen). cDNA was synthesized from 500 ng of total RNA in 20 μl of reaction volume using the High Capacity cDNA Archive Kit (Applied Biosystems). miR-1269a and miR-1269b levels were measured by quantitative PCR using the TaqMan MicroRNA Assay (Applied Biosystems). Gene expression levels were measured by quantitative PCR using the SYBR Green System (Applied Biosystems). All samples were run in triplicates and were repeated three times. The respective miR-1269a and miR-1269b primers and U6 primer were purchased from Applied Biosystems. Other primer sequences include: HOXD10, 5′-GTGCAGGAGAAGGAAAGCAAAG-3′ and 5′-TAACGCTCTTACTGATCTCTAGGC-3′; Smad7, 5'-TGCTCCCATCCTGTGTGTTAAG-3' and 5′-TCAGCCTAGGATGGTACCTTGG-3′; Slug, 5′-CATGCCTGTCATACCACAAC-3′ and 5′-GGTGTCAGATGGAGGAGGG-3′; Snail, 5′-GAGGCGGTGGCAGACTAG-3′ and 5′-GACACATCGGTCAGACCAG-3′; Sox4, 5′-CACATCAAGCGACCCATGAAC-3′ and 5′-CCGGTACTTGTAGTCGGGGTAGT-3′; TGF-β1, 5′-CTCTCCGACCTGCCACAGA-3′ and 5′-AACCTAGATGGGCGCGATCT-3′; TGF-β2, 5′-CCGCCCACTTTCTACAGACCC-3′ and 5′-GCGCTGGGTGGGAGATGTTAA-3′; TGF-β3, 5′-CTGGCCCTGCTGAACTTTG-3′ and 5′-AAGGTGGTGCAAGTGGACAGA-3′; actin, 5′-CGCGAGAAGATGACCCAGAT-3′ and 5′-ACAGCCTGGATAGCAACGTACAT-3′. The expression of each gene was defined from the threshold cycle (Ct), and the relative expression levels were calculated using the 2-ΔΔCt method after normalization to the actin expression level. Lentiviral vector constructs and infection miR-1269a was ectopically expressed by the GFP hsa-miR-1269a Letivector and silenced by the inhibitor hsa-miR-1269a Letivector. These two vectors and the control vectors were ordered from Applied Biological Material. The Smad7 luciferase reporter, with the Smad7 3′UTR in the pMirtarget Vector, was ordered from OriGene. The HOXD10 luciferase reporter, pMIR-D10 UTR, was order from Addgene. miR-1269a-binding sequences in the Smad7 and HOXD10 luciferase reporters were mutated using the QuickChange Site-directed Mutagenesis Kit (Stratagene). To construct the reporter for miR-1269a promoter activity, the miR-1269a promoter sequence was amplified from human genomic DNA and cloned into the pGL4.10 vector (Promega). The putative Sox4-binding site in the miR-1269a promoter sequence was further mutated using the QuickChange Site-directed Mutagenesis Kit (Stratagene). Expression vectors for HOXD10, Smad7, Sox4, Slug and Snail (HOXD10-pcDNA, pBabe-puro-Smad7-HA, pWPXL-Sox4, pBabe-puro-Slug and pBabe-puro-Snail) were ordered from the Addgene. Short hairpin RNA constructs against HOXD10 and Smad7 were ordered from the Sigma. The reporter construct carrying luciferase and mCherry was order from the Addgene. The lentiviral vectors were co-transfected with helper plasmids into 293T cells. The retroviral vectors were transfected into phoenix cells. The viral supernatant was collected 48 h after transfection and was used to infect CRC cells. Luciferase reporter assay To validate the Sox4-binding sites in the miR-1269a promoter, miR-1269a promoter reporter construct with wide-type or mutated Sox4-binding sites was transfected with the pRL-SV40 Renilla luciferase vectors into SW480 and HT29 cells using the LT1 Transfection Reagent (Mirus). To validate whether HOXD10 and Smad7 are direct targets of miR-1269a, HOXD10 and Smad7 luciferase reporter constructs with wide-type or mutated miR-1269a-binding sites were transfected with the pRL-SV40 Renilla luciferase vector into SW480 and HT29 cells. 48 h after transfection, Luciferase assays were performed using the dual luciferase reporter assay system (Promega). Measurements from triplicate transfections were analysed after normalization to the Firefly luciferase activity. Immunofluorescence Cells were grown on glass culture slides (BD Biosciences) and fixed with 4% cold methanol at −20 °C for 10 min. Subsequently, cells were blocked with 10% goat serum for 1 h and incubated with primary antibodies against E-cadherin (24E10, 1:200, Cell Signaling), N-cadherin (1:100, BD Biosciences) and Vimentin (D21H3, 1:100, Cell Signaling) at 4 °C for 1 h and then incubated with Rhodamine Red or Alexa Fluor 488-labelled secondary antibody (Invitrogen) for 1 h at room temperature. After counterstained with DAPI (Invitrogen), the slide was observed under a confocal microscope (Zeiss). Chromatin immunoprecipitation assay ChIP was performed using a ChIP assay kit (Millipore) according to the manufacturer’s instructions. Briefly, SW480 and HT29 cells either infected with a vector-expressing Sox4 or treated with TGF-β1 were incubated in 1% formaldehyde for 10 min at room temperature to crosslink their DNA. The cells were lysed in lysis buffer, sonicated to generate DNA fragments less than 500 base pairs in length and then diluted by tenfolds in ChIP Dilution Buffer. Before immunoprecipitation, nuclear extracts were pre-cleared with 50% protein G–Sepharose slurry, goat normal serum and sheared salmon sperm DNA for 2 h at 4 °C. Anti-Sox4 antibody (H-90, 1:50, Santa Cruz) was then added to form complexes with Sox4 protein and associated chromatin. These immunocomplexes were recovered by protein G–Sepharose beads, and the associated DNA was purified by extraction with phenol/chloroform. PCR Primers 5′-CAGTGGATTGAGTGAGGAAGATTCT-3′ and 5′-TGAGCCCCAGAGTCCAAGAG-3′ for site 1 and primers 5′-CCCTCACAGCAATTTTATAGCATCT-3′ and 5′-TCAAACAAATATGCCAGTCACTTCA-3′ were used to measure the enrichment of the putative Sox4-binding site in the miR-1269a promoter. Western blot Whole-cell lysate was prepared in a lysis buffer (20 mM Tris (pH 7.5), 150 mM NaCl, 1% Nonidet P-40, 0.5% Sodium Deoxycholate, 1 mM EDTA, 0.1% SDS, protease inhibitors). Proteins were first separated by 10% SDS–PAGE and then transferred to a Hybond membrane (Amersham). The membranes were incubated with primary antibodies either anti-E-cadherin (24E10, 1:1000, Cell Signailing), anti-N-cadherin (1:1000, BD Biosciences), anti-HOXD10 (H-80, 1:1000, Santa Cruz), anti-Smad7 (B-8, 1:500, Santa Cruz), anti-Snail (C15D3, 1:1000, Cell Signaling), anti-Slug (C19G7, 1:1000, Cell Signaling), anti-Sox4 (C20, 1:100, Santa Cruz), anti-Phospho-Smad2 (1:1000, Cell Signaling) or anti-β-actin (13E5, 1:1000, Cell Signaling) in 5% milk/TBST buffer (25 mM Tris pH 7.4, 150 mM NaCl, 2.5 mM KCl, 0.1% Triton-X100) overnight, and then probed for 1 h with secondary horseradish peroxidase-conjugated anti-mouse or anti-rabbit IgG (Santa Cruz). After extensive wash with PBST, the target proteins were detected on membrane by enhanced chemiluminescence (Pierce). Full scans of western blots are included in Supplementary Figs11 and 12 . Analysis of Proliferation, migration and invasion SW480 cells were infected with either the control or miR-1269a expression lentiviral vectors. The infection efficiency was measured by GFP expression from the vectors. Cell proliferation under differentiating condition was analysed using the WST-1 Cell Proliferation Reagent (Clontech). Migration assay and invasion assay were performed as previously described. Briefly, 1 × 10 5 cells were plated in the serum-free medium in the upper chamber with the non-coated membrane (24-well insert; pore size, 8 mm; BD Biosciences) for migration assay and with Matrigel-coated membrane (24-well insert; pore size, 8 mm; BD Biosciences) for invasion assay. The lower chamber was filled with medium containing 20% fetal bovine serum. The cells were incubated for 24 h at 37 °C. The cells did not traversed the membrane were removed by a cotton swab and the cells on the lower surface of the membrane were stained with crystal violet and observed under a microscope. In vivo experiments All animal experiments were approved by the Cornell Center for Animal Resources and Education and followed the protocol (2009-0071 and 2010-0100). For subcutaneous injection, 8 × 10 6 cancer cells were injected into the lower back region of 5-week-old female nude mice, with five mice per group. The mice were killed and the tumours were collected and weighed when one of the mice had developed severe tumour burden. For intravenous injection, 2 × 10 6 cancer cells were injected into 5-week-old female NOD/SCID mice, with ten mice per group. The mice were killed and lung/liver metastasis was evaluated when one of them became moribund. For cecum injection, cells were carrying a reporter construct expressing luciferase and mCherry. After FACS sorting, 4 × 10 6 cells were injected into 5-week-old female NOD/SCID mice, with eight mice per group. After injection, luciferase signal was tracked in vivo using the IVIS luciferase imaging system 200 (Xenogen). When one of the mice became moribund, all mice were killed and liver metastases were evaluated based on mCherry signals by an OV100 microscope (Olympus). Immunohistochemistry Lung and liver tissues from mice injected with CRC cells with miR-1269a expression or silencing vectors were removed and fixed in 4% paraformaldehyde overnight. Paraffin-embedded sections were processed for H&E staining. Bioinformatics analysis microRNA expression profiles of CRC tumours at different stages were compared by analysing miRNASeq data from the TCGA COAD data set. A total of 409 samples were grouped according to the AJCC tumour-node-metastasis staging. Stage I (68 samples) and Stage II (162 samples) CRCs were combined to form the early-stage CRC cohort, which was compared with stage IV samples (59 samples) as the late-stage cohort. DESeq was used for differential analysis of the microRNA expression profiling between early- (stage I and II) and late-stage (stage IV) CRC cohorts. Statistical analysis Data were expressed as mean±standard deviation of no smaller than three biological repeats, unless otherwise noted. Student’s t -tests were used for comparisons, with P <0.05 considered significant. Survival curves were estimated using the Kaplan–Meier method and compared using the logrank test. The multivariate analysis was performed with a Cox’s proportional hazards model. Hazard ratios and 95% confidence intervals were derived from the model and the likelihood ratio test was used to compare the groups. How to cite this article : Bu, P. et al. miR-1269 promotes metastasis and forms a positive feedback loop with TGF-β. Nat. Commun. 6:6879 doi: 10.1038/ncomms7879 (2015).